A heavy analogue of the smallest bridgehead alkene stabilized by a base Bicyclo[1.1.0]but-1(2)-ene (BBE), one of the smallest bridgehead alkenes and C 4 H 4 isomers, exists theoretically as a reactive intermediate, but has not been observed experimentally. Here we successfully synthesize the silicon analogue of BBE, tetrasila bicyclo[1.1.0]but-1(2)-ene (Si 4 BBE), in a base-stabilized form. The results of X-ray diffraction analysis and theoretical study indicate that Si 4 BBE predominantly exists as a zwitterionic structure involving a tetrasila homocyclopropenylium cation and a silyl anion rather than a bicyclic structure with a localized highly strained double bond. The reaction of base-stabilized Si 4 BBE with triphenylborane affords the [2+2] cycloadduct of Si 4 BBE and the dimer of an isomer of Si 4 BBE, tetrasila bicyclo[1.1.0]butan-2-ylidene (Si 4 BBY). The facile isomerization between Si 4 BBE and Si 4 BBY is supported by theoretical calculations and trapping reactions. Structure and properties of a heavy analogue of the smallest bridgehead alkene are disclosed. Bridgehead alkenes have a strained doubly bonded carbon at the bridgehead positions in the bicyclic skeleton. Their syntheses, highly strained structures and high reactivities have widely attracted the attention of both theoretical and experimental chemists since the pioneering work of Bredt [1] , [2] , [3] , [4] , [5] . Bicyclo[1.1.0]but-1(2)-ene (BBE, E=C, Fig. 1a ) is a bridgehead alkene with the smallest number of bridge atoms and several possible canonical structures containing a strained double bond [2] , even though BBE has been considered to be an exceptional bridgehead alkene (‘zero-bridge alkene’) because of the lack of a twisted double-bond geometry observed in typical bridgehead alkenes. Although BBE and its derivatives have been proposed as reactive intermediates [6] and theoretically investigated as the isomers of C 4 H 4 molecules present in important fundamental organic molecules such as tetrahedrane and cyclobutadiene [7] , [8] , [9] , [10] , [11] , the synthesis and experimental observation of BBE and its derivatives have not been reported yet. 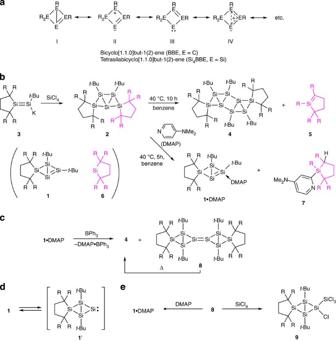Figure 1: Synthesis and reactions of a silicon analogue of the smallest bridgehead alkene. (a) BBE and its silicon analogue (Si4BBE). (b) Synthesis of DMAP-stabilized Si4BEE (1˙DMAP) (R=SiMe3) and the dimer of Si4BBE (4). (c) Reaction of1˙DMAP˙DMAP with triphenylborane (R=SiMe3). (d) A possible equilibrium between Si4BBE1and tetrasilabicyclo[1.1.0]butan-2-ylidene (Si4BBY)1′(R=SiMe3). (e) Reactions of disilene8supporting generation of1and1′(R=SiMe3). Figure 1: Synthesis and reactions of a silicon analogue of the smallest bridgehead alkene. ( a ) BBE and its silicon analogue (Si 4 BBE). ( b ) Synthesis of DMAP-stabilized Si 4 BEE ( 1˙DMAP ) (R=SiMe 3 ) and the dimer of Si 4 BBE ( 4 ). ( c ) Reaction of 1˙DMAP ˙DMAP with triphenylborane (R=SiMe 3 ). ( d ) A possible equilibrium between Si 4 BBE 1 and tetrasilabicyclo[1.1.0]butan-2-ylidene (Si 4 BBY) 1′ (R=SiMe 3 ). ( e ) Reactions of disilene 8 supporting generation of 1 and 1′ (R=SiMe 3 ). Full size image Recently, the silicon analogues of alkenes and structurally related unsaturated organic compounds that have never been experimentally observed or synthesized previously such as pentasila spiropentadiene [12] , tetrasila cyclobutadiene with a planar rhombic charge-separated structure [13] , trisila vinylcarbene [14] , sila vinylidene [15] , Si(0) 2 (ref. 16 ) and isomers of hexasila benzene [17] , [18] have been synthesized as isolable molecules by taking advantage of kinetic stabilization and/or stabilization by base coordination. Their structures and properties have contributed to further understanding of the bonding and structures of organic and heavy main group element π -electron compounds. Among the Si 4 R 4 species, tetrasila tetrahedrane [19] and tetrasila cylobutadiene [13] have been isolated. However, the tetrasila version of BBE (Si 4 BBE, E=Si, Fig. 1a ) has been only theoretically investigated as one of the isomers among the Si 4 R 4 molecules [20] , [21] , whereas it’s detailed molecular and electronic structures and reactivity remain elusive. In this study we report the synthesis of Si 4 BBE 1 , which was stabilized by coordinating to 4-( N , N -dimethylamino)pyridine (DMAP) ( 1·DMAP ). The results of X-ray diffraction (XRD) analysis and theoretical study indicate that Si 4 BBE predominantly exists as a zwitterionic structure containing a tetrasila homocyclopropenylium cation [22] and a silyl anion, rather than a bicyclic structure with a localized double bond. The elimination of DMAP from 1·DMAP with BPh 3 afforded the [2+2] cycloadduct of 1 ( 4 ) and the dimer of tetrasila bicyclo[1.1.0]butan-2-ylidene (Si 4 BBY) 1′ ( 8 ), whose parent molecule was predicted as the global minimum on a Si 4 H 4 surface [20] , [21] . These results indicate a reversible valence isomerization between 1 and 1′ , which was supported by the thermal isomerization of 8 to 4 and reactions of 8 with SiCl 4 and DMAP. Thus, the synthesis, structure, bonding and reactivity of a heavy analogue of the smallest bridgehead alkenes are reported. Thermolysis of hexaalkyltricyclo[2.1.0.0 1,3 ]pentasilane Si 4 BBE 1 was initially suggested to be generated by the thermolysis of hexaalkyltricyclo[2.1.0.0 1,3 ]pentasilane 2 , which was prepared in 63% yield by the reaction of the corresponding potassium trialkyldisilenide 3 (ref. 23 ) with 0.5 equiv. of SiCl 4 ( Figs 1b and 2a ; for the detailed molecular structure of 2 , see Supplementary Information ), similar to the synthesis of Scheschkewitz’s hexaaryl derivative Tip 6 Si 5 2′ (Tip=2,4,6-triisopropylphenyl) [24] . Compound 2 was isolated as reddish purple crystals at ambient temperature. However, heating 2 at 40 °C for 10 h in benzene afforded a mixture of pentacyclo[5.1.0.0 1,6 .0 2,5 .0 3,5 ]octasilane 4 and silene 5 ( Fig. 1b ), whereas Scheschkewitz [24] observed an ion peak assignable to a cluster expansion product with formula Si 7 R 6 during the measurement of the electron ionization mass spectrometry of 2′ . Compound 4 was isolated as orange crystals in 61% yield and identified by nuclear magnetic resonance (NMR) spectroscopy, mass spectrometry (MS), XRD analysis and elemental analysis ( Fig. 2b ). The results of XRD analysis indicate that the silicon skeleton of 4 has a four-membered ring fused by two tetrasila bicyclo[1.1.0]butane units in a syn manner, which is a formal head-to-tail [2+2] cycloadduct of 1 . Notably, the geometry around naked silicon atoms (silicon atoms without substituents), Si3 and Si6 atoms, in 4 are very far from the tetrahedral geometry similar to the naked silicon atoms in 2 and 2′ : For Si3 atom, the angles Si1−Si3−Si2, Si2−Si3−Si4, Si4 –Si3−Si5 and Si1−Si3−Si5 are 60.98(3)°, 57.22(3)°, 94.29(4)° and 163.97(4)°, respectively, and for Si6 atom, the angles Si4−Si6−Si5, Si5−Si6−Si7, Si7−Si6−Si8 and Si4−Si6−Si8 are 94.81(4)°, 57.08(3)°, 60.08(3)° and 162.26(4)°, respectively. The transannular Si2–Si3 and Si6–Si7 bond distances in the terminal tetrasila bicyclo[1.1.0]butane units, 2.4067(11) and 2.4177(11) Å, respectively, are within the range of Si–Si single bond distances. The 29 Si chemical shifts of the naked Si, two ( t -Bu)Si and R H 2 Si nuclei (R H 2 =1,1,4,4-tetrakis(trimethylsilyl)butan-1,4-diyl) are δ −26.8, (−18.4 and −5.5) and 24.6 p.p.m., respectively. As 5 is a thermal isomerization product of dialkylsilylene 6 (ref. 25 ), the generation of 1 and 6 was indicated by the thermolysis of 2 . 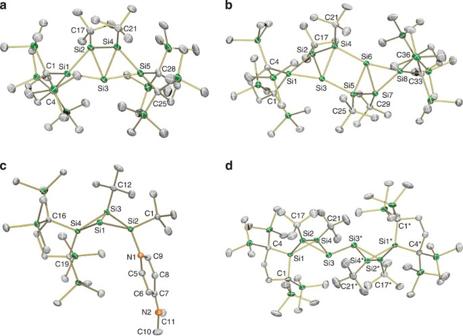Figure 2: Molecular structures of1·DMAPand related compounds as determined by XRD analyses. (a) Tricyclo[2.1.0.01,3]pentasilane2. (b) Pentacyclo[5.1.0.01,6.02,5.03,5]octasilane4(a dimer of Si4BBE1). (c) DMAP-coordinate Si4BBE1·DMAP. (d) Bi(tetrasilabicyclo[1.1.0]butan-2-ylidene)8(a dimer of Si4BBY1′). Thermal ellipsoids are shown at the 50% probability level. Hydrogen atoms are omitted for clarity. Figure 2: Molecular structures of 1·DMAP and related compounds as determined by XRD analyses. ( a ) Tricyclo[2.1.0.0 1,3 ]pentasilane 2 . ( b ) Pentacyclo[5.1.0.0 1,6 .0 2,5 .0 3,5 ]octasilane 4 (a dimer of Si 4 BBE 1 ). ( c ) DMAP-coordinate Si 4 BBE 1·DMAP . ( d ) Bi(tetrasilabicyclo[1.1.0]butan-2-ylidene) 8 (a dimer of Si 4 BBY 1′ ). Thermal ellipsoids are shown at the 50% probability level. Hydrogen atoms are omitted for clarity. Full size image Synthesis of 1·DMAP To obtain monomeric Si 4 BBE 1 , we investigated the thermolysis reaction in the presence of a Lewis base, because coordinating to a Lewis base may stabilize Si 4 BBE 1 , similar to other unsaturated silicon compounds [14] , [15] , [16] , [26] . The reaction of 2 in the presence of 7.6 equiv. of DMAP, which is a typical Lewis base for unsaturated silicon compounds, at 40 °C for 5 h afforded an orange solution. The 1 H NMR spectrum of the mixture indicated the existence of a new compound with 1 and DMAP units together, and 2-silyl-( N , N -dimethylamino)pyridine 7 , which is a product of the reaction of silene 5 with DMAP. Removal of the volatiles from the reaction mixture and repeated recrystallization from hexane at −35 °C and then from benzene at room temperature afforded analytically pure 1·DMAP as orange crystals in 89% yield. The structure of 1·DMAP was determined by NMR spectroscopy, MS spectrometry, XRD analysis and elemental analysis. X-ray analysis of 1·DMAP The results of the XRD analysis of 1·DMAP indicate that the central Si 4 ring has a folded structure with the dihedral angle Si2–Si1–Si3–Si4 of 127.03(2)° ( Fig. 2c ). The nitrogen atom of DMAP coordinates to Si2 atom with the Si2−N1 distance of 1.8764(14) Å, which is moderately longer than the typical Si−N distance (1.71–1.74 Å) [27] . The Si1 atom has no substituent and the Si1−Si3 distance is 2.6215(6) Å, which is considerably longer than those of known tetrasilabicyclo[1.1.0]butanes (2.367–2.412 Å) [28] , [29] , but still shorter than the longest Si−Si distance reported so far (2.697 Å for ( t -Bu) 3 SiSi( t -Bu) 3 ) [30] . The endocyclic Si1–Si2 and Si2–Si3 bond distances, 2.2906(6) and 2.2556(6) Å, respectively, are between the typical Si−Si ( ca . 2.36 Å) [27] and Si=Si bond distances (2.118–2.289 Å) [31] , [32] , and close to those of N -heterocyclic carbene-coordinated cyclotrisilene (trisilacyclopropene) (2.2700(5)Å) [26] , indicating a significant double-bond character in Si1−Si2 and Si2−Si3 bonds. The geometry around Si2 is considerably pyramidalized with the sum of bond angles around Si2 (except the angles involving Si2−N1 bond) of 312.63(4)°, whereas that around Si3 is almost planar with the sum of bond angles around Si3 (except the bond angles involving Si1−Si3 bond), 359.30(4)°. The DMAP moiety exhibits a significant quinoid character. The C5−C6, C8−C9 and C7−N2 bond distances are 1.362(2), 1.359(2) and 1.343(2) Å, respectively, which are shorter than those of the corresponding bonds in free DMAP (1.375(4), 1.381(3) and 1.367(3) Å), whereas the other C−C and C−N bond distances (1.418(2)–1.419(2) and 1.358(2)–1.361(2) Å, respectively) in the pyridine ring of 1·DMAP are longer than those of free DMAP (1.403(3)–1.404(3) and 1.335(4)–1.337(3) Å, respectively) [33] . Theoretical study of 1·DMAP and base-free 1 The comparison of the structural parameters and orbitals between 1·DMAP and base-free 1 obtained by the density functional theory calculations provided further insight into the bonding and structure of 1·DMAP and 1 . The structure of 1·DMAP determined by XRD analysis was well reproduced by the optimized structure of 1·DMAP calculated at the M06-2X/6-31G(d) level ( 1·DMAP opt ) (see Supplementary Fig. 40 ). The dihedral angle, Si2−Si1−Si3−Si4, of 1·DMAP opt is 124.72°, and the Si1−Si2, Si2−Si3, Si1−Si3 and Si1−N1 bond distances are 2.2865, 2.2441, 2.6174 and 1.9368 Å, respectively, which are very close to those of 1·DMAP . The structural parameters of base-free 1 optimized at the same level ( 1 opt ) slightly deviated from those of 1·DMAP opt ( Fig. 3a ). Similar to 1·DMAP , the four-membered ring of 1 opt is folded with the dihedral angle Si4−Si1−Si3−Si2 of 121.89°. The Si1···Si3 distance of 2.849 Å is much longer than the longer end of Si−Si single bond (2.697 Å) [30] and that of 1·DMAP opt (2.620 Å). The endocyclic Si1−Si2 and Si2−Si3 bond distances of 2.228 and 2.207 Å in 1 opt , respectively, are within the range of Si=Si double bond (2.118–2.289 Å) [31] , [32] and shorter than those of 1·DMAP opt (2.286 and 2.244 Å). The bond angle around the unsubstituted Si1 atom (Si4−Si1−Si2) is 85.2°. The geometries around Si2 and Si3 atoms are slightly pyramidalized with the sums of bond angles of 350.24° and 354.98°, respectively. These results indicate that on the coordination of DMAP, the Si1−Si2 and Si2−Si3 bond distances of 1 were elongated (2.286 and 2.244 Å), whereas the Si1−Si3 bond distance was shortened (2.620 Å). A similar elongation of Si=Si double bonds on the coordination of Lewis bases has been reported by Scheschkewitz et al. 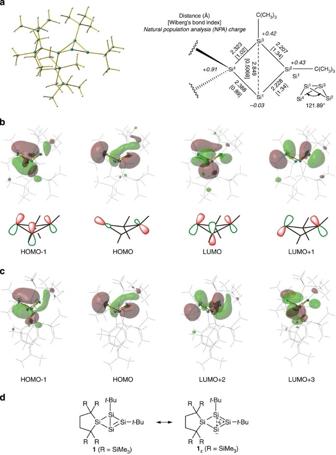Figure 3: Electronic structures of1and1·DMAP. (a) Optimized structure of1(1opt) and selected bond lengths, Wiberg bond indices and the natural charges of1optat the M06-2X/6-31G(d) level. (b) Frontier Kohn–Sham orbitals of1optat the M06-2X/6-31G(d) level. (c) Frontier Kohn–Sham orbitals of1˙DMAPopt. LUMO and LUMO+1 of1˙DMAPoptare the anti-bondingπ-orbitals of pyridine moiety in DMAP. (d) Important canonical structures of1. [26] Figure 3: Electronic structures of 1 and 1·DMAP . ( a ) Optimized structure of 1 ( 1 opt ) and selected bond lengths, Wiberg bond indices and the natural charges of 1 opt at the M06-2X/6-31G(d) level. ( b ) Frontier Kohn–Sham orbitals of 1 opt at the M06-2X/6-31G(d) level. ( c ) Frontier Kohn–Sham orbitals of 1˙DMAP opt . LUMO and LUMO+1 of 1˙DMAP opt are the anti-bonding π -orbitals of pyridine moiety in DMAP. ( d ) Important canonical structures of 1 . Full size image The frontier orbitals of 1 opt and 1·DMAP opt are shown in Fig. 3b,c . The highest occupied molecular orbital (HOMO) of 1 opt is a lone pair orbital on Si1 with the contribution of a p -type orbital on Si3 atom ( Fig. 3b ), which is close to the orbital feature of the interbridgehead bond proposed for all-carbon bicyclo[1.1.0]but-1(2)ene [7] . The HOMO-1 orbital of 1 is an in-phase combination of π (Si1−Si2) orbital and a p -type orbital on Si3 atom. The lowest unoccupied molecular orbital (LUMO) of 1 opt is an out-of-phase combination of π *(Si1−Si2) orbital and a p -type orbital on Si3 atom, and the LUMO+1 is an anti-bonding orbital between Si1 and Si3 atoms. The HOMO-1, LUMO and LUMO+1 orbitals resemble the frontier orbitals of those of tetrasilahomocyclopropenylium cation reported by Sekiguchi et al. [22] , [34] These orbital features indicate that the zwitterionic resonance structure with tetrasilahomocyclopropenylium cation over the Si1–Si2–Si3 atom, and silyl anion on Si1 atoms ( 1 z , Fig. 3d ) contributes significantly to the electronic structure of 1 opt . Very recently, a zwitterionic trisilahomoconjugative compound, a disilaoxaallyl zwitterion was reported by Scheschekwitz et al. [35] The Wiberg bond indices (WBI) of the Si1−Si2 and Si2−Si3 bonds of 1 opt are 1.34 and 1.34, respectively, which are larger than those of Si3−Si4 (1.02) and Si4−Si1 (0.88), respectively, whereas the WBI of Si1−Si3 bond is 0.51, indicating significant bonding interactions between the bridgehead silicon atoms, Si1 and Si3. The natural bonding orbital analysis of 1 opt predicts a three-centred two-electron bond involving Si1 (28.3%), Si2 (35.8%) and Si3 (35.8%) with 1.84 electron and a lone pair on Si1 with 1.88 electron. These results are consistent with the resonance structure of 1 z . The natural population analysis charges of Si1, Si2 and Si3 atoms are −0.02, +0.43 and +0.42, respectively, indicating that Si1−Si2 bond is considerably polar, which is consistent with the formation of head-to-tail cycloadduct 4 . The coordination of DMAP on the Si2 atom of 1 can be rationalized by the positive charge on Si2 and sterically less congested geometry around Si2 compared with those around Si3, indicating that a canonical structure involving disilenylsilylene such as the III of Si 4 BBE in Fig. 1a is a less important contributor. Recently, Scheschkewitz and colleagues [14] reported a base-stabilized disilenylsilylene in which the base coordinates to the two-coordinate silylene centre. At the M06-2X/6-31G(d) level, the coordination of DMAP to 1 opt affording 1·DMAP opt was calculated to be exergonic at 298 K (Δ G 298 K =−39.4 kJ mol −1 ), which is consistent with the experimental observation. The feature of the frontier orbitals of 1·DMAP opt resembles to that of 1 opt ( Fig. 3c ). The WBI of the Si1−Si3 for 1·DMAP opt (0.73) is larger than that for 1 opt (0.51), whereas those of the Si1−Si2 and Si2−Si3 for 1·DMAP opt (1.10 and 1.15) are smaller than those for 1 opt (1.34 and 1.34). The structural change on the coordination of DMAP can be rationalized by the interactions between the lone pair orbital of nitrogen in DMAP and the LUMO of 1 opt involving the bonding interactions between Si1 and Si3, and the anti-bonding interactions between Si1 and Si2, and between Si2 and Si3, resulting in a LUMO+3 orbital. 29 Si NMR spectra of 1·DMAP In benzene- d 6 , three 29 Si resonances arising due to the ring silicon nuclei of 1·DMAP appeared at δ +84.5, +13.3 and −79.8 p.p.m., which were assigned to Si ( t -Bu)(DMAP), Si R H 2 and Si ( t -Bu) silicon nuclei by 2D 1 H- 29 Si NMR HETCOR experiments. No resonance assignable to the naked silicon nuclei was observed probably because of the considerably long relaxation time of the 29 Si nuclei. The assignment of the 29 Si resonances are supported by the density functional theory calculations of 1·DMAP opt (+84.4 ( Si ( t -Bu)(DMAP)), −4.1 (SiR H 2 ) and −105.1 (Si( t -Bu))) and the predicted 29 Si chemical shift of the naked silicon is δ −108.6 p.p.m. These 29 Si resonances indicate that 1·DMAP adopts a structure similar to that observed in the solid state. Elimination of DMAP from 1·DMAP The elimination of DMAP from 1·DMAP was investigated to generate free Si 4 BBE 1 . When a benzene- d 6 solution of 1·DMAP was treated with BPh 3 at room temperature, the colour of the reaction mixture became green, and the NMR spectrum of the mixture indicated the formation of 4 (72% yield) and a disilene with two tetrasila bicyclo[1.1.0]butane skeletons ( 8 ) (8% yield) ( Fig. 1c ). Disilene 8 is the dimer of Si 4 BBY ( 1′ ), which is an isomer of 1 . After keeping the mixture for 48 h at room temperature, 4 was obtained in 78% yield, indicating the isomerization of 8 to 4 . Disilene 8 was isolated as deep blue crystals during the reaction and its structure was determined by XRD analysis, NMR spectroscopy ( Fig. 2d ; for details, see Supplementary Information ). The results indicate the formation of both 1 and 1′ by the reaction of 1·DMAP with BPh 3 , equilibrium between 1 and 1′ ( Fig. 1d ) and the dissociation of disilene 8 into 1′ . These are supported by the reaction of disilene 8 with SiCl 4 and DMAP affording a SiCl 4 adduct of 1′ ( 9 ) and a DMAP adduct of 1 ( 1·DMAP ) ( Fig. 1e ), respectively. The facile isomerization between 1 and 1′ was supported by theoretical calculations. The Si 4 BBY ( 1′ opt ) was optimized as the local minimum at the M06-2X/6-31 G(d) level and 1′ opt is lower in energy by 11.8 kJ mol −1 (298 K) than 1 opt . Similar relative stability for the parent Si 4 H 4 system has been theoretically predicted previously [20] , [21] . A concerted pathway involving the 1,2-migration of SiR H 2 unit from Si1 to Si2 in 1 was predicted for the isomerization of 1 opt to 1′ opt and the calculated Gibbs energy of activation (298 K) for the isomerization was 69.6 kJ mol −1 ( 1′ opt → 1 opt ), which is enough for the reversible isomerization at room temperature to proceed. Although 1′ opt is more stable than 1 opt , the coordination of DMAP to 1 opt (Δ G 298 K =−4.0 kJ mol −1 ) is less exergonic than that for 1 opt (Δ G 298 K =−39.4 kJ mol −1 ) probably because of the reduced Lewis acidity of 1′ resulting from the donation of bridgehead Si–Si bond electrons to the vacant 3 p orbitals of two-coordinate silylene centre. These results are consistent with the observation and isolation of 1·DMAP instead of 1′ ·DMAP. The formation of 4 as the final product in the reaction of 1·DMAP with BPh 3 and the facile dissociation of 8 were also supported by theoretical calculations. The optimized structures of 4 and 8 calculated at the M06-2X level ( 4 opt and 8 opt , respectively, see Supplementary Figs 43 and 44 ) reproduced well structural characteristics of 4 and 8 as determined by XRD analyses. Dimer 4 opt was 53.5 kJ mol −1 more stable than 8 opt and the dimerization of 1 opt into 4 opt was calculated to be considerably exergonic (Δ G 298 K =−106.4 kJ mol −1 ) compared with that of 1′ opt into 8 opt (Δ G 298 K =−52.9 kJ mol −1 ). The calculated bond dissociation enthalpy of the Si=Si bond of disilene 8 opt , 108.5 kJ mol −1 , was much lower than that of tetrasilyldisilene (Me 3 Si) 2 Si=Si(SiMe 3 ) 2 (330.6 kJ mol −1 ) at the M06-2X/6-311G(d) level (see Supplementary Tables 10 and 11 ), but close to that of (Me 5 C 5 )[(Me 3 Si) 2 N]Si=Si[N(SiMe 3 ) 2 ](C 5 Me 5 ) (97.1 kJ mol −1 , at the RI-BP86/TZVP level), which dissociates into the corresponding silylene in solution [36] . The relatively low bond dissociation enthalpy of 8 opt can be mainly attributed to the stabilization of 1′ opt by the donation of bridgehead Si–Si bond electrons to the vacant orbital of two-coordinate silicon centre similar to the π -donation of nitrogen atoms in amino-substituted silylenes. Although other multistep isomerization routes from 8 to 4 or the contribution of DMAP that can accelerate the dissociation of the Si=Si double bond may not be ruled out, a possible mechanism for the formation of 4 from 8 can involve the facile dissociation of 8 to 1′ followed by the isomerization of 1′ to 1 and the dimerization of 1 to afford 4 . A heavy analogue of the smallest bridgehead alkene, Si 4 BBE 1 was successfully synthesized by coordinating to a Lewis base ( 1·DMAP ) and their electronic structure was revealed. The elimination of DMAP from 1·DMAP afforded a mixture of dimers of Si 4 BBE and Si 4 BBY, compounds 4 and 8 . The facile isomerization between compound 1 and its isomer Si 4 BBY 1′ was confirmed both experimentally and theoretically. Synthesis and reactions of Si 4 BBE 1 in this study can be regarded also as an example of contraction and expansion of unsaturated molecular silicon clusters [37] , [38] , [39] , [40] , [41] (termed siliconoids by Scheschkewitz and colleagues [37] ), which have received much attention as possible intermediates of vapour deposition of elemental silicon [42] , [43] . Transformation via elimination of silylene and/or skeletal isomerization may be a fascinating growth route of well-defined silicon clusters showing unique functions. General methods General procedure, materials, experimental details, X-ray analysis and theoretical study in this article are shown in Supplementary Methods . For NMR spectra, Oak Ridge Thermal Ellipsoid Plot (ORTEP) drawings and calculation results of the compounds in this article, see Supplementary Figs 1–31 , Supplementary Figs 32–38 , Supplementary Figs 39–50 and Supplementary Tables 1–13 , respectively. Thermolysis of tricyclo[2.1.0.0 1,3 ]pentasilane 2 To a Schlenk tube (30 ml) equipped with a magnetic stir bar, tricyclo[2.1.0.0 1,3 ]pentasilane 2 (27.5 mg, 0.0291, mmol) and benzene (3 ml) were added. The reaction mixture was heated at 40 °C for 10 h and then benzene was removed in vacuo . Recrystallization of the reaction mixture from hexane at −30 °C afforded pentacyclo[5.1.0.0 1,6 .0 2,5 .0 3,5 ]octasilane 4 as orange crystals (10.2 mg, 0.00893, mmol) in 61% yield. mp: 164 °C (decomposition); 1 H NMR (400 MHz, C 6 D 6 ): δ 0.42 (s, 18H, SiMe 3 ), 0.44 (s, 18H, SiMe 3 ), 0.485 (s, 18H, SiMe 3 ), 0.491 (s, 18H, SiMe 3 ), 1.51 (s, 18H, t -Bu), 1.54 (s, 18H, t -Bu), 1.92–2.20 (m, 8H, CH 2 ); 13 C NMR (100 MHz, C 6 D 6 ): δ 4.39 (SiMe 3 ), 5.16 (SiMe 3 ), 5.23 (SiMe 3 ), 5.58 (SiMe 3 ), 14.2 (C), 17.4 (C), 25.0 (C), 27.4 (C), 32.5 (C( C H 3 ) 3 ), 34.7 (CH 2 ), 35.0 (C( C H 3 ) 3 ), 36.8 (CH 2 ); 29 Si NMR (79 MHz, C 6 D 6 ): δ −26.8 (Si), −18.4 (Si- t -Bu), −5.48 (Si- t -Bu), 3.98 (SiMe 3 ), 4.22 (SiMe 3 ), 4.33 (SiMe 3 ), 4.50 (SiMe 3 ), 24.6 (Si-R H 2 ); HRMS (APCI) ( m / z ): calcd for C 48 H 116 Si 16 , 1,140.5380; found, 1,140.5392; ultraviolet–visible spectra (in hexane): λ max ( ε ) 370 nm (sh, 5,700), 329 nm (sh, 15,000), 268 nm (61,000); analysis (calcd, found for C 48 H 116 Si 16 ): C (50.45, 50.59), H (10.23, 10.31). Reaction of tricyclo[2.1.0.0 1,3 ]pentasilane 2 with DMAP To a Schlenk tube (30 ml) equipped with a magnetic stir bar, tricyclo[2.1.0.0. 1,3 ]pentasilane 2 (142.5 mg, 0.151 mmol), DMAP (140.8 mg, 1.152 mmol) and benzene (10 ml) were added. The reaction mixture was heated at 40 °C for 5 h and then benzene was removed in vacuo . Recrystallization of the reaction mixture from hexane at −35 °C afforded a mixture of DMAP adduct 1·DMAP and excess DMAP. Recrystallization of the resulting reaction mixture from benzene at room temperature afforded pure 1·DMAP as orange crystals (92.8 mg, 0.134 mmol) in 89% yield. The single crystals of 1·DMAP suitable for XRD study were obtained by recrystallization from benzene at room temperature. NMR spectra were measured in the presence of a slight excess of DMAP. mp: 147 °C; 1 H NMR (500 MHz, C 6 D 6 ,): δ 0.03 (s, 9H, SiMe 3 ), 0.38 (s, 9H, SiMe 3 ), 0.61 (s, 9H, SiMe 3 ), 0.83 (s, 9H, SiMe 3 ), 1.48 (s, 9H, t -Bu), 1.62 (s, 9H, t -Bu), 1.88 (s, 6H, Me 2 N), 2.26–2.41 (m, CH 2 (overlapped with the Me of free DMAP)), 2.24 (the Me of free DMAP), 5.52 ( d , J =6.9 Hz, 2H, CH (pyridyl)), 6.11 (the CH of free DMAP), 7.70–8.60 (brs, 2H, CH (pyridyl)), 8.48 (the CH of free DMAP); 13 C NMR (125 MHz, C 6 D 6 ): δ 4.88 (SiMe 3 ), 5.06 (SiMe 3 ), 5.23 (SiMe 3 ), 5.81 (SiMe 3 ), 9.09 (C), 15.5 (C), 22.6 (C), 26.3 (C), 32.1 (C( C H 3 )), 34.8 (C( C H 3 )), 35.1 (CH 2 ), 35.9 (CH 2 ), 105.7 (CH), 155.7 (CH); 29 Si NMR (99 MHz, C 6 D 6 ): δ 1.16 (SiMe 3 ), 2.62 (SiMe 3 ), 4.23 (SiMe 3 ), 4.41 (SiMe 3 ), −79.8 (Si- t -Bu), −84.5 (Si- t -Bu), 13.3 (Si-R H 2 ); 13 C CP/MAS NMR (201 MHz): δ 4.42, 6.28, 9.11, 16.0, 24.3, 26.5, 32.6, 35.5, 41.4, 105.4, 107.2, 146.7, 150.4, 156.5; 29 Si CP/MAS NMR (159 MHz): δ 1.41 (SiMe 3 ), 2.87 (SiMe 3 ), 3.36 (SiMe 3 ), 5.07 (SiMe 3 ), −79.3 (Si- t -Bu), 7.20 (Si-R H 2 ), 78.2 (Si- t -Bu); HRMS (APCI) ( m / z ): ([M] + was missing but [M+H 3 O + ] was found.) calcd for C 31 H 71 N 2 OSi 8 , 711.3715; found, 711.3718; analysis (calcd, found for C 31 H 68 N 2 Si 8 ): C (53.68, 53.35), H (9.88, 9.72), N (4.04, 4.17). In the 13 C NMR spectrum in C 6 D 6 solution, the signals due to the CH 3 and aromatic carbons of coordinating DMAP were not observed. In the 29 Si NMR spectrum, both in the solution and solid states the signal due to two-coordinate silicon nuclei (Si1) was not observed. How to cite this article : Iwamoto, T. et al. A heavy analogue of the smallest bridgehead alkene stabilized by a base. Nat. Commun. 5:5353 doi: 10.1038/ncomms6353 (2014). Accession codes : The X-ray crystallographic coordinates for structures reported in this study have been deposited at the Cambridge Crystallographic Data Centre (CCDC), under deposition numbers CCDC 1007442 ( 1·DMAP ), CCDC 1007443 ( 2 ·(benzene) 0.5 ), CCDC 1007444 ( 2 ·(2,3-dimethy-1,3-butadiene) 0.5 ), CCDC 1007445 ( 4 ·(benzene)), CCDC 1007446 ( 7 ), CCDC 1007447 ( 8 ) and CCDC 1007448 ( 9 ). These data can be obtained free of charge from The Cambridge Crystallographic Data Centre via www.ccdc.cam.ac.uk/data_request/cif .